Three-dimensional broadband ground-plane cloak made of metamaterials Since invisibility cloaks were first suggested by transformation optics theory, there has been much work on the theoretical analysis and design of various types and a few experimental verifications at microwave and optical frequencies within two-dimensional limits. Here, we realize the first practical implementation of a fully 3D broadband and low-loss ground-plane cloak at microwave frequencies. The cloak, realized by drilling inhomogeneous holes in multi-layered dielectric plates, can conceal a 3D object located under a curved conducting plane from all viewing angles by imitating the reflection of a flat conducting plane. We also designed and realized, using non-resonant metamaterials, a high-gain lens antenna that can produce narrow-beam plane waves in the near-field region in a broad frequency band. The antenna constitutes the transmitter of the measurement system and is essential for the measurement of cloaking behaviour. Invisibility cloaks had only been a figment of human imagination until the appearance of optical transformation theory [1] . Transformation optics has provided the conceptual design of novel and complicated electromagnetic and optical devices by controlling the paths of wave propagation [2] , [3] . The routes of electromagnetic waves can be controlled by choosing the material parameters through artificial metamaterials [4] . When the incoming electromagnetic waves are guided to propagate around a metamaterial shell region and return to their original propagation paths without interacting with the object inside, the metamaterial shell is called a free-space invisibility cloak [1] . Mathematically, the invisibility cloak is used to compress the object into a point. In recent years, transformation optics has been applied to analyse and design a large variety of cloaks theoretically [5] , [6] , [7] , [8] . However, only a few experiments have been conducted. The first experimental demonstration of a reduced invisibility cloak was realized using resonant metamaterials in the microwave frequency [9] , which has a narrow frequency band with a relatively large loss. Owing to the extreme requirement for the electric permittivity and magnetic permeability, the realization of full cloak is still unavailable, although several new designs have been presented to mitigate the requirement [10] , [11] , [12] , [13] . In view of the difficulty to realize the free-space cloaks, a ground-plane cloak (or carpet cloak) was proposed based on the optical transformation, which can hide any objects under a ground plane covered by the metamaterial carpet [14] . Mathematically, the ground-plane cloak crushes the hidden object to a conducting sheet instead of a point. Physically, the object hidden under the ground-plane cloak appears as a flat conducting sheet. Followed by the theoretical prediction by Li and Pendry [14] , the first experimental demonstration of the ground-plane cloak was realized in the microwave frequencies [15] . As the ground-plane cloak does not require singular values for the material parameters, I-shaped non-resonant metamaterial structures were used to construct the cloak, which results in good cloaking properties of broadband and low loss [15] . Such promising properties have also been found in the experiments of optical ground-plane cloaks [16] , [17] . Recently, a modification of the experiment has been carried out to reduce the size of ground-plane cloaks in the microwave frequencies [18] . However, all the above-mentioned experiments on the invisibility cloaks have been in the two-dimensional (2D) limit. More specifically, the cloaking devices were two-dimensional and the experiments were performed in a 2D planar waveguide [9] , [15] , [16] , [17] , [18] . Hence, the above cloaks were only effective to the transverse-electric (TE)-polarized incident waves. Besides the transformation optics approach, other techniques have also been proposed to reduce the scattering cross section of various objects [19] , [20] , [21] . For example, in recent theoretical and numerical studies, homogeneous and isotropic plasmonic covers have been used to dramatically reduce the scattered fields by a given object based on the scattering compensation [19] , [20] ; the transmission-line cloak and the metal-plate cloak have been realized to study the cloaking behaviour of a metal object from an electromagnetic pulse inside a rectangular waveguide [21] . In this article, we present the first practical realization of a fully 3D broadband ground-plane cloak in the microwave frequency, which can conceal a 3D object located under a curved conducting plane from all viewing angles by imitating the reflection of a flat conducting plane. Following a similar theoretical procedure to that of 2D cloak, we obtain the constitutive parameter distributions for the 3D cloak. We design the 3D cloak using inhomogeneous isotropic dielectric materials, which are realized by drilling inhomogeneous holes in layered dielectric plates. Hence, the 3D cloak has broadband and low loss. To measure the cloaking properties of the 3D cloak, we also designed and realized a high-gain lens antenna using non-resonant metamaterials as the transmitter of the measurement system, which can produce narrow-beam plane waves in the near-field region in a broad frequency band. The experimental results show good performance of the 3D cloak for different polarized incident waves. The 3D ground-plane cloak has important potential applications in the microwave frequencies, such as to hide aircrafts on the airport and automobiles on the road from the radar detection. The proposed design and realization methods can be easily extended to the optical frequencies to produce fully 3D optical ground-plane cloaks. Design of the fully 3D ground-plane cloak In the description of 2D ground-plane (or carpet) cloaks [14] , [15] , [16] , [17] , [18] , the incident waves were restricted to a single plane to which the electric field is perpendicular (TE-polarized incidence). Hence, only the cloak parameters in this plane were required, yielding a 2D problem (see Fig. 2 in reference Li and Pendry [14] , Fig. 1c in Liu et al . [15] and Fig. 1b in Ma et al . [18] ). From the optical transformation theory, the 2D ground-plane cloaks have good cloaking performance to all incident angles. If we suppose that the plane is in the Cartesian x–z coordinates ( Fig. 1c,d ), the incident angles are elevation angles. By rotating the 2D cloak around the z axis, we generate a 3D cylindrical ground-plane cloak ( Supplementary Fig. S1a ). Hence, the 3D cloak parameters can be easily obtained by rotating the available 2D cloak parameters. Figure 2: Unit cells used in the design of the cloak and the relation of geometry to electric field polarization. 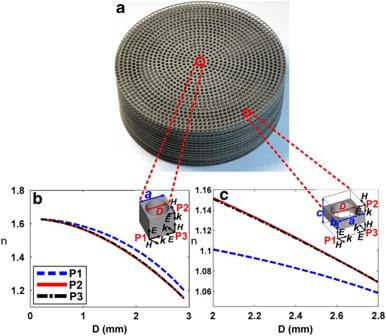Figure 2: Unit cells used in the design of the cloak and the relation of geometry to electric field polarization. (a) The designed ground-plane cloak. (b) The 3×3×3 mm3drilled-hole unit cell, in whicha=3 mm, and the relations between effective index of refraction and unit-cell geometry for different polarized incident electric fields at 10 GHz. P1, P2 and P3 are three orthogonal polarizations,EandHare the electric and magnetic field andkis the wave vector of the incident radiation. (c) The 3×3×1 mm3drilled-hole unit cell, in whicha=3 mm,b=3 mm andc=1 mm, and the relations between effective index of refraction and unit-cell geometry for different polarized incident electric fields at 10 GHz. ( a ) The designed ground-plane cloak. ( b ) The 3×3×3 mm 3 drilled-hole unit cell, in which a =3 mm, and the relations between effective index of refraction and unit-cell geometry for different polarized incident electric fields at 10 GHz. P1, P2 and P3 are three orthogonal polarizations, E and H are the electric and magnetic field and k is the wave vector of the incident radiation. 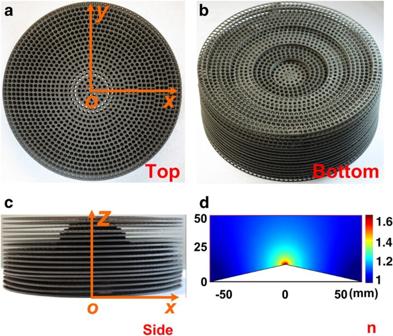( c ) The 3×3×1 mm 3 drilled-hole unit cell, in which a =3 mm, b =3 mm and c =1 mm, and the relations between effective index of refraction and unit-cell geometry for different polarized incident electric fields at 10 GHz. Figure 1: Three-dimensional microwave ground-plane cloak and its refractive index distribution. (a) Top view of the cloak. (b) Bottom view of the cloak. (c) Side view of the cloak. (d) The distribution of refractive index in thex–zplane. The material parameters of the whole cloak are obtained by rotating thex- toz-plane pattern around thezaxis. Full size image Figure 1: Three-dimensional microwave ground-plane cloak and its refractive index distribution. ( a ) Top view of the cloak. ( b ) Bottom view of the cloak. ( c ) Side view of the cloak. ( d ) The distribution of refractive index in the x–z plane. The material parameters of the whole cloak are obtained by rotating the x - to z -plane pattern around the z axis. Full size image In the presented 3D ground-plane cloak, we choose the parameter distribution in the x–z plane as that for the 2D cloak given in ref. 18 . Then, we get the full 3D parameter distributions by rotating it around the z axis. Comparing with the original designs [14] , [15] , the 2D ground-plane cloak described in reference Ma et al . [18] has a much smaller size (about four times smaller). The designed 3D cloak is resided in the free space (that is, the background is air), which is suitable for real cases for potential applications in the microwave frequency. In our design, conformal mapping was used to obtain the refractive indices of the cloak, and the anisotropic factor is 1.07. The required 3D material parameters are shown in Figure 1d and Supplementary Figure S1b , whose refractive indices range from 1 to 1.63, and hence they can be easily realized using non-resonant metamaterials [15] or the conventional dielectric materials [16] . Here, we generate the 3D ground-plane cloak by drilling inhomogeneous holes in multi-layered dielectric plates. Photographs of the fabricated 3D cloak sample are illustrated in Figure 1a–c . The outline shape of the cloak is a 3D cylinder whose height and bottom radius are 51 mm and 62.5 mm, respectively. On the bottom of the cloak, the cloaked region (perturbation) is a cone-shaped metallic bump whose bottom radius and height are 62.5 mm and 13 mm, respectively, as shown in Figure 1d . The 3D cloak is fabricated using multi-layered drilled-hole dielectric plates ( Fig. 2a ), which are made of polytetrafluoroethylene and glass fibre (F4B), with the relative permittivity of 2.65 and loss tangent of 0.001. The standard height of F4B dielectric plate is 1 mm. To realize the drilled-hole metamaterials, two different-size unit cells are used to design the 3D cloak: 3×3×3 mm 3 and 3×3×1 mm 3 , as shown in Figure 2b and c , respectively. Using a well-established retrieval process [22] , the effective values of relative permittivity, permeability, characteristic impedance and refractive index for above-mentioned unit cells can be achieved by numerical simulations. For the 3×3×3 mm 3 cubic unit cells (a=3 mm), the diameter of the drilled hole is D . By varying D , the effective indices of refraction change gradually. Figure 2b shows the relationship between the effective indices of refraction and the size D at 10 GHz, in which three orthogonal polarizations of incident waves (P1, P2, P3) have been considered. We observe clearly that the same electromagnetic responses are obtained for the polarizations P2 and P3, with a little difference for the polarization P1. When D varies from 0 to 2.9 mm, the refractive index changes from 1.63 to 1.15 for the P2 and P3 polarizations, whereas it changes from 1.63 to 1.20 for the P1 polarization. The small difference can be ignored and the 3×3×3 mm 3 unit cells can be approximately regarded as isotropic. Similarly, the 3×3×1 mm 3 unit cells also have the approximately isotropic property, as shown in Figure 2c . If D varies from 2 to 2.8 mm, the refractive index changes from 1.15 to 1.07. On the basis of the above-mentioned analysis, the part of the 3D cloak whose refractive indices are larger than 1.15 is fabricated using the 3×3×3 mm 3 unit cells with different-diameter holes, and the other part whose refractive indices are smaller than 1.15 is fabricated using the 3×3×1 mm 3 unit cells with different-diameter holes. In realization, the 3×3×3 mm 3 unit cells are obtained by stacking three-layered standard F4B dielectric plates together and the 3×3×1 mm 3 unit cells are obtained from a single standard F4B plate. The fabricated 3D cloak is illustrated in Figure 1a–c , which contains 17 layers of drilled-hole F4B plates. The detailed realization of the 3D cloak is presented in Methods and is shown in Supplementary Figure S2 . Continuous-material equivalence In the designs presented above, we make use of the drilled-hole metamaterials to realize the continuous-material properties required by the 3D cloak. To illustrate the equivalence between continuous materials and actual drilled-hole metamaterials, the best way is to simulate the ideal 3D cloak composed of continuous materials and the experimental 3D cloak composed of drilled-hole metamaterials simultaneously and to compare their electromagnetic properties. However, the full-wave simulation of the experimental 3D cloak is impossible using the current computer, owing to the extremely large memory requirement and computing time. Instead, we make full-wave simulations to a dielectric plate, which can be regarded as one layer of the 3D cloak. Consider a circular dielectric plate whose radius and thickness are 62.5 mm and 3 mm, respectively. The dielectric plate is composed of continuous materials and the distribution of refractive index is given by n =(2.6– r 2 / R 2 ) 1/2 , in which 0< r < R and R =62.5 mm. When the continuous-material plate is inserted in a planar waveguide, it is equivalent to a TE-polarized 2D problem. We perform a full-wave simulation using the finite-element method to investigate the electromagnetic properties. 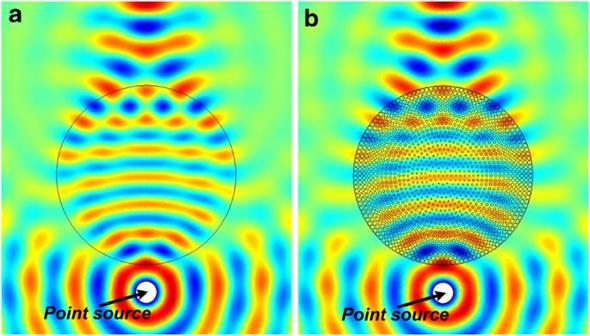Figure 3: Full-wave simulation results of electric fields inside and outside the metamaterials. The calculations are performed for the circular continuous-material and drilled-hole metamaterial plates under the excitation of a 2D point source at 10 GHz. Both plates have a radius of 62.5 mm and a thickness of 3 mm, and are placed in a planar waveguide. Hence, the simulations can be performed using 2D models (TE polarization). (a) Continuous-material plate. (b) Drilled-hole metamaterial plate. Figure 3a illustrates the electric-field distribution inside and outside the continuous-material plate under the excitation of a 2D point source at 10 GHz. Figure 3: Full-wave simulation results of electric fields inside and outside the metamaterials. The calculations are performed for the circular continuous-material and drilled-hole metamaterial plates under the excitation of a 2D point source at 10 GHz. Both plates have a radius of 62.5 mm and a thickness of 3 mm, and are placed in a planar waveguide. Hence, the simulations can be performed using 2D models (TE polarization). ( a ) Continuous-material plate. ( b ) Drilled-hole metamaterial plate. Full size image On the other hand, we make use of the drilled-hole metamaterials to realize the continuous-material plate using the 3×3×3 mm 3 unit cells, in which totally 1,310 inhomogenous holes are drilled on a 3 mm-thick F4B dielectric plate with a relative permittivity of 2.65. From Figure 2b (P1 polarization), when the hole diameter varies from 0.6 mm (for the central hole) to 2.7 mm (for the boundary holes), we can obtain the same distribution of the effective index of refraction as that of the continuous-material plate. Under the same condition, we perform the full-wave simulation of the drilled-hole structure using finite-element method, and the simulation result of electric fields inside and outside the drilled-hole metamaterial plate is shown in Figure 3b . Excellent agreement is observed for electric fields both inside and outside the plate by comparing Figure 3a and b . Hence, the drilled-hole metamaterials have nearly the same electromagnetic properties as the continuous materials. In the other words, the drilled-hole metamaterials used in the experimental 3D cloak do have the bulk material behaviours that are expected by an ideal 3D cloak. Experiment setup To verify the cloaking performance of the designed 3D ground-plane cloak, we set up an experiment system in a fully anechoic chamber to measure the scattering behaviours of a flat ground plane, the ground plane with the cone-shaped perturbation and the ground plane with the perturbation and cloak. In experiments, the ground plane is a copper plate with the size of 55×40 cm 2 . 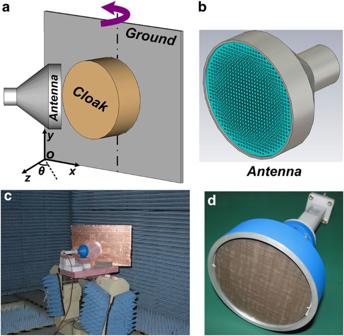Figure 4: Measurement system of the 3D ground-plane cloak. A metamaterial lens antenna is used to transmit a narrow-beam plane wave in the near-field region, and a normal X-band rectangular horn antenna is used to receive the far-field scattered electric fields. (a) The demonstration of measurement. (b) The sketch of the metamaterial gradient index lens antenna. The green surface is made of metamaterials. (c) The actual measurement system in a fully anechoic chamber. (d) The photograph of the metamaterial antenna. Figure 4a–c shows the measurement system. A metamaterial lens antenna is used to transmit a narrow-beam plane wave in the near-field region, and a normal X-band rectangular horn antenna located in the other side of the anechoic chamber is used to receive the far-region scattered fields. The bricks used to support the antenna, ground plane and 3D cloak are made of foam, which has nearly the same index of refraction as the air, and hence has little effect on measurements. Owing to the rotating symmetrical property of the 3D cloak, we perform the measurements in the x–z plane ( φ =0, see Supplementary Fig. S1 ). The incident direction of the metamaterial transmitter is arbitrarily chosen as θ =−45° with respect to the ground and is fixed, and the whole system rotates around the y axis to get varying receiving directions ( θ =−90 to 90°). Figure 4: Measurement system of the 3D ground-plane cloak. A metamaterial lens antenna is used to transmit a narrow-beam plane wave in the near-field region, and a normal X-band rectangular horn antenna is used to receive the far-field scattered electric fields. ( a ) The demonstration of measurement. ( b ) The sketch of the metamaterial gradient index lens antenna. The green surface is made of metamaterials. ( c ) The actual measurement system in a fully anechoic chamber. ( d ) The photograph of the metamaterial antenna. Full size image In experiments, the metamaterial transmitter has an important role. As the measured objects (ground plane, perturbation and 3D cloak) have relatively small sizes, the reflecting and scattering properties cannot be well captured under the illumination of conventional horn antenna in the far-field region, which radiates the approximate plane wave with wide beam. Here, we designed a gradient index metamaterial lens antenna ( Fig. 4b ) fed by a circular horn and rectangular waveguide ( Fig. 4d ) as the transmitter, in which the lens aperture is 98 mm. As the metamaterial antenna can produce a narrow-beam plane wave in the near-field region, it is an excellent candidate to measure the reflecting property of the ground plane with finite size and the scattering property of the bump. The metamaterial lens was made of inhomogeneous closed-square rings (CSR), which are non-resonant metamaterial unit cells. By adjusting the size of CSR, we are able to control the refractive index to achieve the gradient index lens. Owing to the non-resonant nature, the lens antenna has a broadband, which works from 8 GHz to 12 GHz, covering the whole X-band. Simulation and experimental results show that the lens antenna radiates perfect plane waves and has high gains in both E-plane and H-plane. The detailed design, simulations and measurements of the metamaterial lens antenna are presented in Methods and are shown in Supplementary Figures S3–S7 . 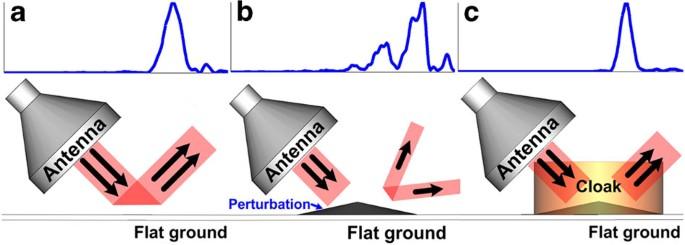Figure 5: Three situations for measurements and simulations and the predicted far-field patterns. (a) The flat ground plane, with a single-peak reflection at the mirror-reflecting direction of the incident wave. (b) The ground plane with a cone-shaped metallic perturbation, with multi-peak reflections. (c) The ground plane with both perturbation and 3D cloak, with a single-peak reflection at the mirror-reflecting direction of the incident wave. The electric field amplitude in the top half of the panels is normalized to unity. Observation of cloaking effect To observe the cloaking effect clearly, three kinds of measurements are taken in the experiments: the flat ground plane, the ground plane with cone-shaped perturbation (the bump) and the ground plane with both perturbation and 3D cloak, as illustrated in Figure 5a–c , respectively. We expect that the measured scattering property of the ground plane with perturbation ( Fig. 5b ) is significantly distinct to that of the ground plane ( Fig. 5a ), whereas the measured scattering property of the ground plane with both perturbation and cloak ( Fig. 5c ) is nearly the same as that of ground plane. Figure 5: Three situations for measurements and simulations and the predicted far-field patterns. ( a ) The flat ground plane, with a single-peak reflection at the mirror-reflecting direction of the incident wave. ( b ) The ground plane with a cone-shaped metallic perturbation, with multi-peak reflections. ( c ) The ground plane with both perturbation and 3D cloak, with a single-peak reflection at the mirror-reflecting direction of the incident wave. The electric field amplitude in the top half of the panels is normalized to unity. Full size image Two polarizations of incident waves have been considered in the measurement: the incident electric field is parallel to the x–z plane (parallel polarization) and perpendicular to the x–z plane (perpendicular polarization). Such polarizations can be achieved by adjusting the feeding rectangular waveguide of the metamaterial lens. We have measured the scattered electric fields of the flat ground plane, the ground plane with perturbation and the plane with both perturbation and cloak at 9 GHz, 10 GHz and 12 GHz, respectively. Numerical simulations of the three situations are also provided, in which the 3D cloak is modelled by continuous materials. All simulations were performed using the full-wave commercial software (Microwave Studio, Computer Simulation Technology). We remark that the metamaterial lens antenna was considered in the full-wave simulations, in which the gradient index lens is also modelled by continuous materials. 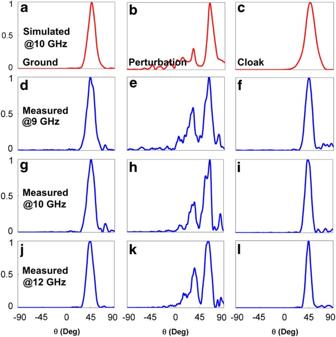Figure 6: The simulated and measured electric fields in the far region. The fields are shown at different frequencies under the incidence of parallel-polarized electric field emitted from the metamaterial lens antenna.θ isthe incidence angle, whereas the electric field amplitudes are normalized to unity. (a–c) Simulated results for the three situations at 10 GHz. (d–f) Measured results for the three situations at 9 GHz. (g–i) Measured results for the three situations at 10 GHz. (j–l) Measured results for the three situations at 12 GHz. For the parallel-polarization incidence, the simulated and measured results are shown in Figure 6 . Good agreements between measurements ( Fig. 6g–i ) and simulations ( Fig. 6a–c ) are clearly observed at 10 GHz, which confirms the equivalence of the drilled-hole metamaterials and the continuous materials. As the 3D cloak is made of layered F4B dielectric plates, it is expected to exhibit a large frequency range of operation. This was confirmed by our measurements in the frequency range 9–12 GHz. From Figure 6a, d, g and j , the flat ground plane produces a single-peak reflection at the mirror-reflecting direction of the incident wave. However, the presence of the cone-shaped metallic perturbation generates considerable scattering with multi-peak reflections, as shown in Figure 6b, e, h and k . When the perturbation is covered by the designed 3D cloak, however, the single-peak reflection is restored as if the ground plane were flat, as shown in Figure 6c, f, i and l . It is obvious that good cloaking effects are achieved using the 3D cloak in a broad frequency band for the parallel polarization. 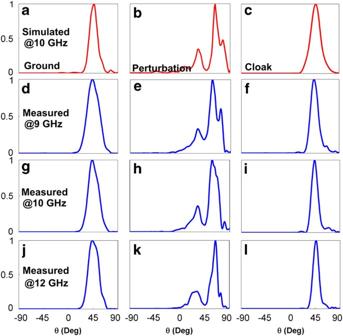Figure 7: The simulated and measured electric fields in the far region. The fields are shown at different frequencies under the incidence of perpendicular-polarized electric field emitted from the metamaterial lens antenna.θ isthe incidence angle, whereas the electric field amplitudes are normalized to unity. (a–c) Simulated results for the three situations at 10 GHz. (d–f) Measured results for the three situations at 9 GHz. (g–i) Measured results for the three situations at 10 GHz. (j–l) Measured results for the three situations at 12 GHz. Figure 7 illustrates the simulated and measured results for the three situations as the incident electric field is perpendicular-polarized, and similarly good cloaking performance are observed. Figure 6: The simulated and measured electric fields in the far region. The fields are shown at different frequencies under the incidence of parallel-polarized electric field emitted from the metamaterial lens antenna. θ is the incidence angle, whereas the electric field amplitudes are normalized to unity. ( a–c ) Simulated results for the three situations at 10 GHz. ( d–f ) Measured results for the three situations at 9 GHz. ( g–i ) Measured results for the three situations at 10 GHz. ( j–l ) Measured results for the three situations at 12 GHz. Full size image Figure 7: The simulated and measured electric fields in the far region. The fields are shown at different frequencies under the incidence of perpendicular-polarized electric field emitted from the metamaterial lens antenna. θ is the incidence angle, whereas the electric field amplitudes are normalized to unity. ( a–c ) Simulated results for the three situations at 10 GHz. ( d–f ) Measured results for the three situations at 9 GHz. ( g–i ) Measured results for the three situations at 10 GHz. ( j–l ) Measured results for the three situations at 12 GHz. Full size image On the basis of the theoretical prediction and experiments on 2D ground-plane cloaks [14] , [15] , [16] , [17] , [18] , we designed, fabricated and measured the first fully 3D ground-plane cloak in the microwave frequency. The presented 3D cloak is generated by rotating the 2D cloak around the z axis, and hence the distribution of refractive index is varied in the 3D space. This is the first cloaking device that is independent of the incident elevation angle θ (similar to the 2D case), the incident azimuth angle φ (owing to the rotating symmetry) and the polarization of incident wave in a broad frequency band. The 3D cloak presented here was designed using inhomogeneous isotropic dielectric materials, whose refractive index ranged from 1 to 1.63, and was fabricated by drilling inhomogeneous holes in multi-layered commercial F4B dielectric plates with the relative permittivity of 2.65. Hence, the cloak has a broadband and low loss in the microwave frequency. The full-wave simulation results showed that the drilled-hole metamaterials have nearly the same electromagnetic properties as the continuous materials (see Fig. 3 ). As a consequence, the artificial metamaterials used in the experimental 3D cloak do have the bulk material behaviours that are expected. Owing to the easy fabrication with isotropic material, the fully 3D cloak can be directly extended to the optical frequency using the technique presented in reference Gabrielli et al . [17] . Note added in proof : While this article was under consideration, another implementation of a 3D cloak was published [23] . Geometry of 3D ground-plane cloak The 3D ground-plane cloak in the Cartesian coordinate system is illustrated in Supplementary Figure S1a , in which the z axis is perpendicular to the ground plane. The elevation angle θ is defined as the angle from the radius vector to the z axis, and the azimuth angle φ is defined as the angle from the projection of the radius vector on the x–y plane to the x axis. The 3D ground-plane cloak is generated by rotating the 2D ground-plane cloak on the x–y plane around the z axis. Hence, the 3D cloak is cylindrically symmetrical with respect to the azimuth angle φ . Fabrication of 3D ground-plane cloak The 3D ground-plane cloak is composed of two kinds of unit cells: 3×3×3 mm 3 and 3×3×1 mm 3 , as shown in Figure 2b and c , respectively. The cloak is fabricated using multi-layered drilled-hole F4B dielectric plates. In total, the designed cloak has 17 layers, and in each layer some regions are generated using the 3×3×3 mm 3 unit cells (region I in Supplementary Fig. S2 ) and some regions are generated using the 3×3×1 mm 3 unit cells (region II in Supplementary Fig. S2 ). According to the well-established retrieval process, we can obtain the diameter of each drilled hole at any location for all layers to achieve the required index of refraction. The thickness of standard F4B plates used here is 1 mm, with the relative permittivity of 2.65 and loss tangent of 0.001. As an example, we consider the generation of the top layer, as shown in Supplementary Figure S2a,b . The 3×3×1 mm 3 unit cells are easily fabricated using a single F4B plate. For the region with 3×3×3 mm 3 unit cells (region I), we fabricate two more identical F4B plates with the same drilled holes (see Supplementary Fig. S2a ) and stick them on region I to get the required thicknesses of 3 mm (see Supplementary Fig. S2b ). Similarly, the other 16 layers are designed and fabricated in the same way. Then, we stack such 17 layers together to obtain the full 3D ground-plane cloak, as illustrated in Supplementary Figure S2c . Metamaterial lens antenna We adopted a gradient index lens antenna to generate the narrow-beam plane waves in the near-field region. On the basis of the geometrical optics, the spherical waves excited by a point source can be transformed into plane waves when propagating through a properly designed circularly planar lens [24] , [25] , [26] , as shown in Supplementary Figure S3 . To make such a transformation, the index of refraction should have gradient distribution along the aperture as in which, 0< r < R , n 0 is a positive real constant, S is the distance between lens and feeding source and R and T are radius and thickness of the lens. To minimize reflections from the lens, impedance-matching layers (IMLs) between the lens and air were designed [27] . The final sketch of the lens antenna is shown in Supplementary Figure S4a . In the design, n 0 =1.86, T =27 mm, S =48 mm, R =49 mm, d 1 =25 mm, d 2 =98 mm, t 1 =30 mm, t 2 =37.5 mm, t 3 =6 mm and t 4 =15 mm. The Phase-correcting abilities of the lens with and without IMLs have been shown to be the same [27] . The distributions of refractive indices for the core and IMLs are given in Supplementary Figure S4b , in which the refractive index of the core varies from 2.17 to 1.13, and the refractive index of IMLs varies from 1.47 to 1.06, from the lens centre ( r =0) to the lens edge ( r = R ). In designing the lens antenna, non-resonant CSR metamaterial structures were used [27] , which were printed on the F4B dielectric substrate with the thickness of 0.5 mm, the relative permittivity of 2.65 and the loss tangent of 0.001. Supplementary Figure S5 shows the relationship between the effective material parameters of CSR and the dimension d at 10 GHz, in which the edge length of CSR is a =3 mm and the line width is w =0.2 mm. When d is increased from 0.8 to 2.8 mm, there is nearly no magnetic response for CSR, and the corresponding effective index of refraction varies gradually from 1.16 to 2.41. Hence, the gradient index lens can be achieved by arranging a series of CSRs with different dimensions [27] . On the basis of the above design, the metamaterial lens antenna was fabricated using the gradient index CSR structures, as illustrated in Supplementary Figure S6 [27] . The designed antenna has good properties. Supplementary Figure S7a,b shows the simulated electric-field distributions of the antenna in the E-plane and H-plane at 10 GHz. We clearly observe that the lens antenna can generate narrow-beam plane waves in the near-field region. The measured far-field radiation patterns in the E- and H-planes are illustrated in Supplementary Figure S7c,d . The measured results show that the designed antenna has high directivity and low side lobes in the whole X-band. We remark that the E-plane corresponds to the parallel polarization and the H-plane corresponds to the perpendicular polarization. How to cite this article: Ma, H.F. et al . Three-dimensional broadband ground-plane cloak made of metamaterials. Nat. Commun. 1:21 doi: 10.1038/ncomms1023 (2010).